Identifying the preferred RNA motifs and chemotypes that interact by probing millions of combinations RNA is an important therapeutic target but information about RNA–ligand interactions is limited. Here, we report a screening method that probes over 3,000,000 combinations of RNA motif-small molecule interactions to identify the privileged RNA structures and chemical spaces that interact. Specifically, a small molecule library biased for binding RNA was probed for binding to over 70,000 unique RNA motifs in a high throughput solution-based screen. The RNA motifs that specifically bind each small molecule were identified by microarray-based selection. In this library-versus-library or multidimensional combinatorial screening approach, hairpin loops (among a variety of RNA motifs) were the preferred RNA motif space that binds small molecules. Furthermore, it was shown that indole, 2-phenyl indole, 2-phenyl benzimidazole and pyridinium chemotypes allow for specific recognition of RNA motifs. As targeting RNA with small molecules is an extremely challenging area, these studies provide new information on RNA–ligand interactions that has many potential uses. RNA has diverse functions in cellular biology including encoding and translating protein, regulating the amount of protein expressed under different cellular conditions, and many others [1] , [2] , [3] , [4] . In addition, RNA has been used as an artificial molecular switch to control cellular events such as RNA splicing and gene expression [5] . Because of this, RNA is an attractive target for small molecules that serve as chemical genetics probes or therapeutics [6] , [7] , as effectors of artificial gene circuits or as analytical tools [5] , [8] . Various studies have identified small molecules that bind RNA [6] , [9] , [10] ; however, the available information is sparse compared with the structural diversity of RNA in the transcriptome. One method that has been used to identify RNA structures that bind small molecules is systematic evolution of ligands by exponential enrichment (SELEX). In a SELEX experiment, aptamers (derived from an RNA library with a randomized region typically of >20 nucleotides) is identified that binds a small molecule with high affinity and specificity [11] , [12] . As the selected RNA is rather large, it is difficult to find it in genomic RNAs. However, there have been some excellent and notable cases in which the output of SELEX has been found in a biologically relevant RNA [13] , [14] . A more common use of aptamer–small molecule interactions has been in the development of engineered cellular switches [5] . Another approach used to identify RNA–ligand interactions is high-throughput screening (HTS) [6] , [7] . In this approach, a single validated RNA probe or drug target is screened for binding to libraries of small molecules. Screening can be accomplished by using various techniques including structure-activity relationships (SAR) by NMR spectroscopy [15] , SAR by mass spectrometry [16] , [17] , among others [18] , [19] . Screening endeavors to find compounds that bind RNA, however, have much lower hit rates when compared with identifying small molecules that bind protein. Often, the hits identified are not specific for the RNA probed [6] . In an effort to develop a bottom-up rather than the traditional top-down approach to target RNA, we previously reported a method that merges the advantages of SELEX and of high throughput small molecule screening [20] , [21] . This method probes chemical and RNA motif spaces simultaneously to identify selective interactions that can be used to target RNA. Termed 2-dimensional combinatorial screening (2DCS), a library of small molecules is probed for binding to libraries of small RNA motifs that are likely to be present in a biologically important RNA. By using selection to identify the RNA motifs that bind each small molecule, the optimal RNA motif–small molecule partners are identified. These interactions are mined against RNA secondary structures in the transcriptome to design small molecules against a functionally important or toxic RNA. This approach has led to the development of small molecules that potently target several RNAs that contribute to disease, such as the myotonic dystrophies and Huntington's disease [22] , [23] , [24] , [25] . In this report, we describe the development of an approach that allows for the facile identification of RNA motif–ligand interactions by merging solution-based HTS with microarray-based selection of the RNA motifs that bind a small molecule. This approach is high throughput and high content in that it probes millions of potential RNA motif–small molecule partners. Using this method, it was determined that members of a small molecule library have a significant bias for binding to RNA hairpin loops over thousands of other structures including internal loops, bulges and base pairs. Analysis of the chemical space of the active small molecules reveals chemotypes that bias small molecules for recognition of RNA. This approach may have implications for the design of small molecules that modulate RNA function, which is important yet an extremely challenging area. HTS and microarray-based selections We previously described a multidimensional combinatorial screening (MDCS) platform (also termed library-versus-library screening) that was developed to identify the optimal RNA motifs from a library of discrete secondary structures that bind small molecules ( Figs 1b and 2 ). Termed 2DCS, a microarray of small molecules is hybridized with a library of RNA motifs, such as internal loops, under conditions of high stringency [20] , [21] . The randomized region of the RNA libraries is intentionally small ( Fig. 2 ) such that the structures have a high probability of occurring in biological RNAs [20] , [21] . The boundmotifs are collected from the microarray via excision, amplified by RT–PCR, and identified by cloning and sequencing. 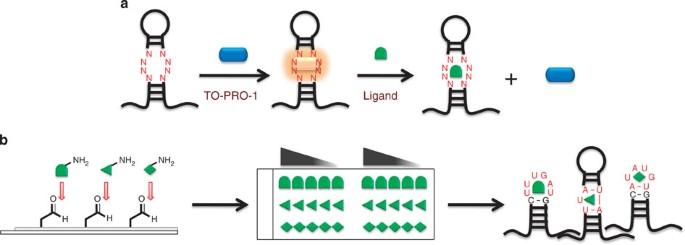Figure 1: The general procedure used to merge solution-based small molecule HTS with microarray-based selection of RNAs that bind ligands. (a) Ligands are identified that bind to RNA motif libraries by using a TO-PRO-1 dye-displacement assay. (b) The RNA motifs that bind to each arrayed ligand are identified by microarray-based selection20,21. Briefly, ligands identified that bind RNA from the dye-displacement assay are conjugated to microarray surfaces and hybridized with RNA motif libraries under highly stringent conditions. Bound RNAs are collected from the array by manual excision and sequenced. Figure 1: The general procedure used to merge solution-based small molecule HTS with microarray-based selection of RNAs that bind ligands. ( a ) Ligands are identified that bind to RNA motif libraries by using a TO-PRO-1 dye-displacement assay. ( b ) The RNA motifs that bind to each arrayed ligand are identified by microarray-based selection [20] , [21] . Briefly, ligands identified that bind RNA from the dye-displacement assay are conjugated to microarray surfaces and hybridized with RNA motif libraries under highly stringent conditions. Bound RNAs are collected from the array by manual excision and sequenced. 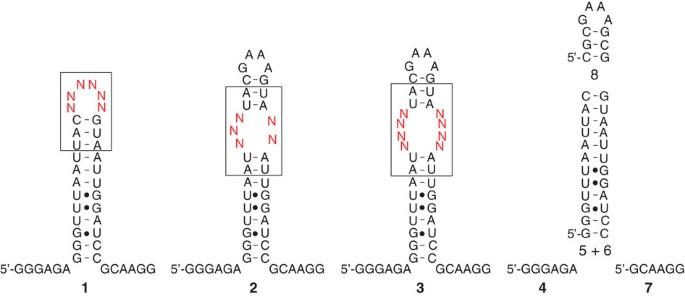Figure 2: The structures of the RNA motif libraries and the competitor oligonucleotides used in this study. N represents an equimolar mixture of A, C, G and U. RNA motif libraries1–3contain 4,096, 1,024 and 65,536 members, respectively. Oligonucleotides4–8are used to compete off interactions that are common to all library members during selection experiments. Full size image Figure 2: The structures of the RNA motif libraries and the competitor oligonucleotides used in this study. N represents an equimolar mixture of A, C, G and U. RNA motif libraries 1 – 3 contain 4,096, 1,024 and 65,536 members, respectively. Oligonucleotides 4 – 8 are used to compete off interactions that are common to all library members during selection experiments. Full size image The direct microarray approach, however, is not amenable to more traditional small molecule screens. For example, high-throughput screens that are completed under the Molecular Libraries Program at the National Institutes of Health (NIH) use solution-based screening to identify hit compounds that bind a target. Thus, to gain access to such resources and to increase the number of chemotypes and RNA motifs that are known to interact, we developed an approach that merges more standard high-throughput, solution-based screens with microarray-based selection strategies ( Fig. 1 ). We then used this method to determine the features in RNA motifs (hairpins, internal loops and bulges) and the features in small molecules that impart high affinity, selective binding. Specifically, the approach employs a solution-based dye-displacement screening assay to identify small molecules that bind RNA motif libraries ( Fig. 1 ). The small molecules identified from this screen are then subjected to the previously described microarray-based MDCS selection. Selection of a dye for solution-based HTS To complete a high-throughput screen of RNA–ligand interactions, a read-out of binding is required. Previous studies have shown that dyes with emission properties that significantly change upon binding RNA can be used as probes in fluorescent indicator displacement assays to identify small molecules that bind nucleic acids [26] , [27] , [28] , [29] , [30] . Examples include: a 2,7-disubstituted 9H-xanthen-9-one, or X2S, which has been used to study the binding of a library of pharmaceutically active compounds (LOPAC) to HIV Rev-responsive element RNA [30] ; TO-PRO-1, which has been used to study the binding of small molecule ligands to a variety of RNAs [28] ; and thiazole orange (TO), which has been used to study the binding of threading intercalators to RNA [29] . To identify a dye that is optimal for our HTS approach, we investigated the fluorescence properties of four unrelated dyes (TO-PRO-1, X2S, ethidium bromide and SYBR green II) in the presence and absence of RNA library 1 , which displays hairpin loops ( Fig. 2 ). The fluorescence intensity of TO-PRO-1, ethidium bromide and SYBR green II increases in the presence of 1 , whereas the fluorescence intensity of X2S decreases. Table 1 summarizes the EC 50 for 1 , or the concentration of 1 at which the half maximal change in fluorescence is observed, and the sensitivity, defined as the percentage change in fluorescence intensity at the EC 50 , for all four dyes. In summary, TO-PRO-1 binds 1 with the lowest EC 50 (550 nM) and with excellent sensitivity (~450%). The EC 50 's for ethidium bromide and X2S are slightly higher (1,400 and 850 nM, respectively); however, their sensitivities are significantly decreased (~ninefold). Although the sensitivity of SYBR green II is the highest of the four dyes, no saturable binding to 1 was observed. (Also see Supplementary Fig. S1 ). Table 1 EC 50 and sensitivities of dyes for RNA library 1 . Full size table The fluorescence properties of dyes can also be affected by the presence of small molecules. We therefore completed two sets of experiments: dye was incubated individually with members of a small molecule library; and, dye was incubated individually with members of a small molecule library and 1 . The results of these experiments are shown in Supplementary Figs S2–S5 . Even though X2S and ethidium bromide bind 1 with relatively low EC 50 's, their emission properties are significantly affected by the presence of small molecules, decreasing the signal to noise ratio. SYBR green II is less affected by the presence of small molecules globally; however, this is not the case for a subset of the compounds screened. In contrast, there is very little variability in the fluorescence intensity of TO-PRO-1 in the presence of small molecules. Thus, TO-PRO-1 was used to identify the features in RNA motifs and small molecules that impart binding affinity and selectivity. Solution-based HTS The general strategy of the HTS approach is illustrated in Fig. 1 . Three RNA motif libraries were used that include a 4,096-member 6-nucleotide hairpin library ( 1 ), a 1,024-member 3×2-nucleotide asymmetric internal loop library ( 2 ) and a 65,536-member 4×4-nucleotide symmetric internal loop library ( 3 ) ( Fig. 2 ). Each of these RNA motif libraries was chosen because they display small RNA motifs that are highly abundant in cellular RNAs. Thus, the specific small molecule–RNA motif partners identified from this approach could be utilized as lead ligands to modulate RNA function, provided a biologically important RNA that contains a targetable motif can be identified. Advances in RNA structure prediction and annotation from sequence provide relatively simple approaches to identify targetable motifs that are present in RNAs [31] , [32] , [33] . In our initial studies, the three RNA motif libraries ( 1 – 3 , Fig. 2 ) were screened for binding to small molecules that are biased for binding to RNA by using a TO-PRO-1 displacement assay in 384-well plate ( Fig. 1a ). Previously, it was shown that chemical similarity-based virtual screening can be used to define a population of small molecules that are biased for binding to RNA [34] , [35] . Various studies have identified privileged scaffolds that bind RNA including benzimidazoles [22] , [24] , [34] , [36] , [37] , [38] , [39] , pentamidine [35] , [40] , [41] , [42] , [43] and 4′,6-diamidino-2-phenylindole (DAPI) [23] , [34] , [41] , some of which are bioactive. Thus, a library of small molecules based on these scaffolds and therefore biased for binding RNA was constructed (43 compounds; Supplementary Table S1 ) [22] , [23] . The compounds were generally restricted to contain an amino or imino group such that they could be anchored site-specifically onto aldehyde-functionalized agarose microarrays for selection of RNA motifs [21] , [44] , [45] . The RNA libraries were incubated with TO-PRO-1, and then the ligand of interest was added at 100 μM. If the ligand binds the RNA target, then a decrease in fluorescence intensity is observed due to dye displacement. Using this method, eight compounds that bind 1–3 were identified, affording a hit rate of 19% ( Fig. 3a ). One compound is similar to pentamidine (pentamidine-like, PL ; PL-1 ), four compounds are Hoechst-like ( HL ; HL-1 , HL-2 , HL-3 and HL-4 ) and three compounds are DAPI-like ( DL ; DL-1 , DL-2 and DL-3 ) ( Fig. 3a ). To ensure that ligands were not aggregating (forming self-structure) and then displacing TO-PRO-1, the screen was repeated in the presence of Igepal detergent. No significant change in TO-PRO-1 displacement was observed for all compounds except for two, indicating that ligand aggregation is generally not occurring ( Supplementary Fig. S6 ). (Neither of the two compounds was one of the four ligands for which the preferred RNA motif space was determined). 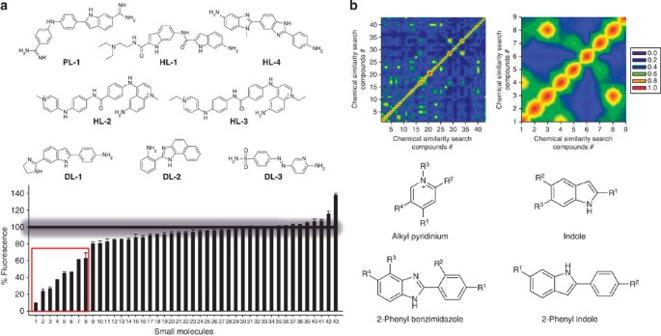Figure 3: Solution-based screen and chemoinformatic analysis of the hit compounds. (a) Solution-based screen identifies small molecules that bind1–3. Top, the structures of the top eight ligands identified. Bottom, data for screening the entire library for binding1. A '% Fluorescence' of 100% indicates that the compound does not displace TO-PRO-1, whereas '% Fluorescence' below 100% indicates that the small molecule binds the RNA and displaces TO-PRO-1. (b) Chemoinformatic analysis of the hit compounds. Top left, two-dimensional plot of the Tanimoto scores for each small molecule as compared with every library member. Top, right, a close-up view of the plot to the left for the top eight hit compounds. Bottom, results of common scaffold analysis of the top eight hit ligands reveals features in chemical space that facilitate RNA binding. Figure 3: Solution-based screen and chemoinformatic analysis of the hit compounds. ( a ) Solution-based screen identifies small molecules that bind 1 – 3 . Top, the structures of the top eight ligands identified. Bottom, data for screening the entire library for binding 1 . A '% Fluorescence' of 100% indicates that the compound does not displace TO-PRO-1, whereas '% Fluorescence' below 100% indicates that the small molecule binds the RNA and displaces TO-PRO-1. ( b ) Chemoinformatic analysis of the hit compounds. Top left, two-dimensional plot of the Tanimoto scores for each small molecule as compared with every library member. Top, right, a close-up view of the plot to the left for the top eight hit compounds. Bottom, results of common scaffold analysis of the top eight hit ligands reveals features in chemical space that facilitate RNA binding. Full size image To assess the quality of the hit rate of our RNA-focused library relative to a library that is unbiased for binding RNA and to demonstrate the scalability of the screening method, we applied the TO-PRO-1 displacement assay to the 1,280-member LOPAC ( Supplementary Figs S7–S9 ). The LOPAC library provided only 13 hits, or a hit rate of 1.0%. Thus, by using a library enriched in chemotypes for binding RNA, a 19-fold increase in the hit rate is obtained. Chemoinformatic analysis identifies privileged chemotypes The chemotypes in the entire library of compounds, including the eight hit compounds, were then analyzed for structural similarity ( Fig. 3b ). The analysis was completed by comparing the shape-based similarity (Tanimoto) scores [46] of every compound to each other. Tanimoto scores range from 0–1.0 and quantitatively assign the shape similarity between two compounds (where a score of 1.0 indicates complete shape similarity). When considering the entire library, some compounds are highly similar to each other; however, most have only modest or moderate similarity. For the hit compounds, there is an increase in their similarity to each other. The average Tanimoto similarity score of each compound in the library to all the others is 0.29±0.12, whereas the average Tanimoto similarity score between the eight hit compounds is 0.43±0.15. Thus, there is a slight enrichment in the features that are similar within the hit compounds; that is, the hit compounds are more similar to each other than the entire library is similar to itself. In addition, the structures of the eight hit compounds ( Fig. 3a ) were analyzed for common scaffolds according to the method of Clark and Labute [47] . The common scaffolds include indole, 2-phenyl indole, 2-phenyl benzimidazole and pyridinium groups ( Fig. 3b ). Information on the chemotypes that are biased for selective recognition of RNA is important for the development of RNA-focused small molecule libraries. Thus, small molecule collections that contain chemotypes that allow for selective RNA recognition should have a higher hit rate when screened for binding to RNA targets compared with non-RNA focused libraries, such as LOPAC. Microarray-based selection of RNA-ligand interactions The solution-based screen identifies lead small molecules that bind RNA. However, hit compounds can be selected that bind to the randomized region or to the constant regions in the RNA motif libraries ( Fig. 2 ). To identify the small molecules that bind to the randomized region in the RNA, a secondary screening assay is completed. In this secondary assay, the eight hit compounds from the TO-PRO-1 displacement assay were conjugated onto a microarray surface and probed for binding to RNA motifs under highly stringent conditions. Specifically, arrays were incubated simultaneously with 32 P-labeled RNA motif libraries 1 – 3 in the presence of a large excess (>1,000-fold) of unlabeled competitor oligonucleotides 4 – 8 and d(AT) 11 and d(GC) 11 ( Fig. 2 ). Thus, the RNA motifs that bind to each small molecule are selected, and small molecules that bind the constant regions are eliminated. Good signal is observed for PL-1 , HL-1 , HL-2 and DL-1 , indicating that they bind specifically to the randomized regions in 1 – 3 even under highly stringent conditions ( Fig. 4a ). In contrast, HL-3 , DL-2 , DL-3 and HL-4 failed to give signal over background ( Fig. 4a ). These compounds are unable to bind the randomized regions under highly stringent conditions and likely bind to the constant regions. 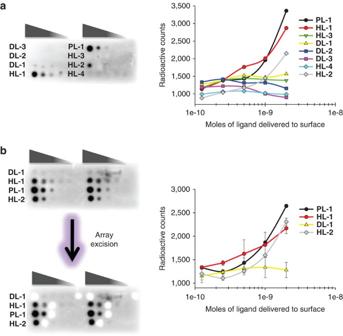Figure 4: MDCS selection of RNA motifs that bind to small molecules. (a) Image of a microarray displaying the eight hit compounds after hybridization with radioactively labeled1–3and unlabeled4–8(Fig. 2)20,21,48, and a plot of the corresponding data. OnlyPL-1,HL-1,HL-2andDL-1bind to1–3under these highly stringent conditions and were subjected to microarray-based selections. (b) Image of a microarray displayingPL-1,HL-1,HL-2andDL-1after hybridization with radioactively labeled1–3and unlabeled competitors4–8, and a plot of the corresponding data. The error bars are the standard deviations. Figure 4: MDCS selection of RNA motifs that bind to small molecules. ( a ) Image of a microarray displaying the eight hit compounds after hybridization with radioactively labeled 1 – 3 and unlabeled 4 – 8 ( Fig. 2 ) [20] , [21] , [48] , and a plot of the corresponding data. Only PL-1 , HL-1 , HL-2 and DL-1 bind to 1 – 3 under these highly stringent conditions and were subjected to microarray-based selections. ( b ) Image of a microarray displaying PL-1 , HL-1 , HL-2 and DL-1 after hybridization with radioactively labeled 1 – 3 and unlabeled competitors 4 – 8 , and a plot of the corresponding data. The error bars are the standard deviations. Full size image To ensure the interactions of PL-1 , HL-1 , HL-2 and DL-1 are specific to the RNA libraries, arrays displaying PL-1 , HL-1 , HL-2 and DL-1 were hybridized with 1 in the presence of a large excess of tRNA (500 times the number of moles of compound delivered to the surface and 8,000 times the concentration of 1 ; Supplementary Fig. S10 ). Excellent signal was still observed for all compounds. Subsequently, compounds PL-1 , HL-1 , HL-2 and DL-1 were subjected to microarray-based selection using the oligonucleotides competitors described above ( Fig. 2 ) [20] , [21] , [48] . Three rounds of selection were completed before sequencing the RNA motifs that bind each ligand. As shown in Fig. 4b , RNAs that bind to each compound were cleanly excised from the microarray surface. RT–PCR amplification, cloning and sequencing identified the bound RNAs. Identification of privileged RNA space An initial statistical analysis was completed to determine if the small molecules are biased for binding one particular RNA motif library. Due to the differences in the number of library members in each library and biases that may be introduced during RT–PCR amplification or cloning, the starting population of RNAs applied to the microarray surface was subjected to RT–PCR amplification, cloning and sequencing (see Supplementary Figs S12–S15 for the sequences of selected RNAs). The representation of each library in the sequencing data was used as baseline in the statistical analysis of the results from our selection (see Supplementary Table S2 ). Our statistical analysis is completed using a population comparison. For example, the proportion of hairpin loops in the sequencing data of the starting library is compared with the proportion of hairpin loops in the selected RNAs. This difference is then used to calculate statistical significance, reported as a Z -score. The results of this analysis are present in Table 2 . All four small molecules have a strong bias for binding to RNA hairpins that are derived from 1 (positive Z obs ) and a bias against members in libraries 2 and 3 (negative Z obs ). These general trends were also observed when the individual selections were analyzed. Table 2 Statistical analysis of selected RNAs for binding PL-1 , HL-1 , HL-2 and DL-1. * Full size table To precisely define the RNA motif space preference for each ligand, the selected RNA sequences were analyzed by using a statistical approach [49] , [50] . In this approach, the populations of RNA motifs that comprise the starting library are compiled, and the occurrence rate of each feature in the library is compared with the occurrence rate of that feature in the selected RNA motifs. By comparing these two populations, the relative enrichment for a specific feature in RNA motif space for binding to a ligand can be computed. This enrichment is assigned a statistical significance or a Z -score and the corresponding two-tailed P -value. Statistical analysis was completed using a method that we describe as structure-activity relationships through sequencing (StARTS) [49] , [51] . Briefly, the RNA-Privileged Space Predictor program (RNA-PSP, v. 2.0) [50] extracts the nucleotides that are derived from the randomized positions in selected RNAs. The sequences and the features within them are analyzed to determine statistical biases relative to the entire library. The individual features are assigned a Z -score. Each RNA can have multiple privileged features for binding a ligand. Thus, the Z -scores for all features that occur with ≥95% confidence are summed to afford the sum Z -score [49] , [50] , [51] . Previous studies have shown that the RNA motifs with the highest sum Z -scores bind to a ligand with the highest affinity, whereas ones with lower sum Z -scores bind more weakly [49] , [51] . A Venn diagram was derived based on the statistically significant features that have a confidence level of ≥99% in RNA hairpin loops selected to bind PL-1 , HL-1 , HL-2 and DL-1 (when four bases are defined and two are N's; Supplementary Fig. S11 ). These features most commonly have AU, UA or AG steps. Compounds PL-1 , HL-1 and DL-1 have overlapping RNA hairpin loop space that includes many different orientations of AU or UA steps. RNA motif space that is unique for HL-1 , HL-2 and DL-1 generally have G's in hairpin loops, whereas unique space for PL-1 typically has UU or AA steps. The affinities of RNA–ligand interactions The RNA motifs with the highest sum Z -scores for binding each ligand are shown in Fig. 5 and were studied for binding to the corresponding small molecule ligand (see Supplementary Figs S16–S19 for characterization of these small molecules). (The secondary structures shown in Fig. 5 were predicted by free energy minimization using the RNAstructure program [31] .) As each small molecule used in this particular MDCS study is fluorescent, binding constants were determined in solution by measuring the change in fluorescence intensity of the small molecule as a function of RNA concentration. In addition, the affinities of the ligands for the starting libraries were also determined to measure the enrichment in affinity that the selection strategy provides. 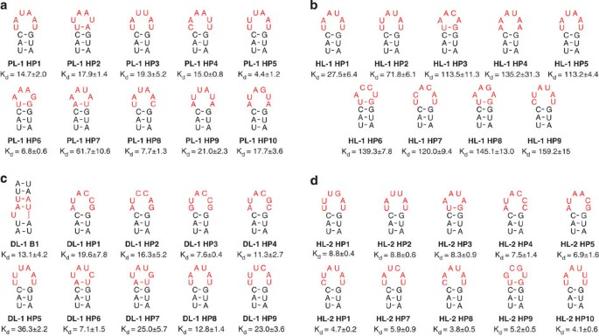Figure 5: Secondary structures and affinities of the selected RNA motif–ligand interactions. The secondary structures shown were predicted by free energy minimization using the RNAstructure program31. The RNA motif–ligand partners that were subjected to binding assays were predicted to have the highest affinities based on analysis by structure-activity relationships through sequencing (StARTS)49,50,51. The red letters in the secondary structures indicate nucleotides that are derived from the randomized region of the libraries; the secondary structure shown is from the boxed nucleotides inFig. 2. All dissociation constants (Kd) are reported in micromolar.PL-1,HL-1,HL-2andDL-1do not bind oligonucleotide8(Fig. 2; GAAA tetraloop) or the starting libraries1–3(Kd>200 μM). (a) The RNA motifs selected to bindPL-1. (b) The RNA motifs selected to bindHL-1. (c) The RNA motifs selected to bindDL-1. (d) The RNA motifs selected to bindHL-2. In the RNA identifiers, 'B' indicates a bulge, whereas 'HP' indicates a hairpin. Each experiment was completed in triplicate, and the error bars are the standard deviations. Figure 5: Secondary structures and affinities of the selected RNA motif–ligand interactions. The secondary structures shown were predicted by free energy minimization using the RNAstructure program [31] . The RNA motif–ligand partners that were subjected to binding assays were predicted to have the highest affinities based on analysis by structure-activity relationships through sequencing (StARTS) [49] , [50] , [51] . The red letters in the secondary structures indicate nucleotides that are derived from the randomized region of the libraries; the secondary structure shown is from the boxed nucleotides in Fig. 2 . All dissociation constants (K d ) are reported in micromolar. PL-1 , HL-1 , HL-2 and DL-1 do not bind oligonucleotide 8 ( Fig. 2 ; GAAA tetraloop) or the starting libraries 1 – 3 (K d >200 μM). ( a ) The RNA motifs selected to bind PL-1 . ( b ) The RNA motifs selected to bind HL-1 . ( c ) The RNA motifs selected to bind DL-1 . ( d ) The RNA motifs selected to bind HL-2 . In the RNA identifiers, ' B ' indicates a bulge, whereas ' HP ' indicates a hairpin. Each experiment was completed in triplicate, and the error bars are the standard deviations. Full size image Saturable binding was observed for each of the selected RNA motifs. The range of affinities observed for each small molecule is different. For example, PL-1 , DL-1 and HL-2 have dissociation constants in the low micromolar range, whereas HL-1 binds slightly weaker to its selected RNAs with affinities ranging from 30 to 160 μM ( Fig. 5 ). In contrast, no saturable binding was observed for any of the ligands with the starting RNA motif libraries 1 – 3 ( Fig. 2 ), indicating K d 's>>200 μM. Oligonucleotide 8 , which mimics the GAAA hairpin in RNA libraries 2 and 3 ( Fig. 2 and Supplementary Figs S22–S25 ), has a K d >>200 μM, whereas tRNA has a K d 2,400 μM ( Supplementary Fig. S27 ). The affinities of the selected RNA motifs for the corresponding small molecules in these studies are weaker than those previously observed for aminoglycoside derivatives used in 2DCS selections [20] , [21] . However, they are similar to those observed for a series of benzimidazoles [51] , including a rigid benzimidazole derivative that binds to and modulates the function of the hepatitis C virus internal ribosomal entry site (IRES) [36] . This compound binds to an asymmetric internal loop in IRES with mid-micromolar affinity and inhibits propagation [36] . As our initial screen was completed in solution, it is possible that binding affinity is affected by conjugation to the slide surface. That is, immobilization of the compound through the amino or imino group could affect molecular recognition. Therefore, we studied the binding of a DL-1 derivative that mimics the structure of the compound when displayed on an array surface to four RNAs selected to bind DL-1 ( DL-1 B1 , DL-1 HP1 , DL-1 HP2 and DL1-HP3 ; Fig. 5 and Supplementary Fig. S28 ). The free amine in DL-1 was reacted with benzaldehyde via reductive amination to afford DL-1 benzyl ( Supplementary Figs S20–S21 ). For DL-HP1 and DL-HP2 , the affinities for DL-1 and DL-1 benzyl are the same or within error. The change in the affinities of DL-1 B1 and DL-1 HP2 for the two compounds is modest (13±4 and 37±7 μM for DL-1 B1 ; 8±1 and 34±6 μM for DL-1 HP3 ). Similar results were previously observed for the RNA motifs that prefer to bind 6′- N -5-hexynoate kanamycin A. The affinities of 6′- N -5-hexynoate kanamycin A and kanamycin A were comparable. [20] Interestingly, no signal for HL-3 was observed on the microarray despite the fact that it is very similar to HL-2 . To determine if this observation was an artifact of the microarray selection, the affinity of HL-3 for the RNAs selected for HL-2 were determined as described above. No binding of HL-3 was observed to any of the RNAs ( Supplementary Fig. S26 ), in good agreement with the observations from the microarray experiment. Furthermore, these studies indicate that subtle differences in chemical structure can significantly affect RNA-binding affinity. Recent studies have established that RNA has critical and varied roles in disease. Small molecules that bind these RNAs and modulate function/toxicity could serve as chemical genetics probes or therapeutics. Lead compounds could be developed based on the preferences of small molecules for RNA secondary structural motifs. At present, however, such information is sparse and has hampered the development of compounds targeting RNA. Herein, we have utilized a modified version of 2DCS to quickly identify chemotypes in small molecules that bind RNA and the RNA motif preferences for binding small molecules. There are immediate uses for this information. First, transcriptomes can be mined to identify RNAs that have the targetable motifs identified from our studies. These ligands could then be tested for modulating the function of the corresponding RNAs. Second, chemically diverse small molecule libraries that are biased for binding RNA could be constructed using the privileged chemotypes defined herein. Libraries that are currently screened for binding RNA are generally biased for modulating protein function, thus yielding much lower hit rates for RNA targets. Also, we will use this approach to screen larger, more chemically diverse small molecule libraries, which will undoubtedly define additional chemotypes that impart affinity for RNA recognition and additional RNA motifs that are preferred by small molecules. General instrumentation and procedures Please refer to the Supplementary Method for more detail on instrumentation, chemical, nucleic acids and general procedure for PCR amplification of DNA templates encoding selected RNAs, transcription and purification of selected RNAs. HTS of RNA–ligand interactions Before screening, the EC 50 's of TO-PRO-1 to the RNA motif libraries were determined. Briefly, the RNA library of interest ( 1 – 3 , Fig. 2 ) was folded in 1× Screening Buffer 1 (SB1; 8 mM Na 2 HPO 4 , pH 7.0, 185 mM NaCl, 0.1 mM EDTA) at 60 °C for 5 min followed by slowly cooling to room temperature on the bench top. BSA was then added to a final concentration of 40 μg ml −1 to afford 1× SB2. The RNA was titrated into 100 nM TO-PRO1 prepared in 1× SB2, and the fluorescence intensity was measured after each addition using an excitation wavelength of 485 nm and an emission wavelength of 528 nm. The resulting curves were fit to a one-site binding model. The EC 50 's are: 1 544±67 nM; 2 239±38 nM; and 3 558±54 nM. The concentration of RNA library that corresponded to the EC 50 's for binding TO-PRO-1 were used in the TO-PRO-1 displacement assay. The RNA libraries ( 1 , 2 or 3 ) were folded as described above. TO-PRO-1 was then added to a final concentration of 100 nM. The RNA/TO-PRO-1 mixture was incubated at room temperature for 15 min. Then, 10 μl of this solution was dispensed into each well of a black 384-well plate (Greiner Low-Volume 784076) using an Aurora Discovery FRD-1B liquid dispenser. A 100-nl aliquot of a 10 mM stock of each small molecule was pinned into each well using Biomek NXP Laboratory Automation Workstation that was equipped with a 384-pin head. The solution was incubated at room temperature for 15 min. Fluorescence intensity was measured on an Envision 2104 Multilabel Plate Reader (Perkin Elmer) with an excitation wavelength of 485/14 nm, an emission wavelength of 528/25 and a 505-nm cutoff mirror. The change in fluorescence was normalized to a percentage response (%Res) according to the equation 1: where I represents the fluorescence intensity of each sample, Ĩ −ve represents the median of the fluorescence intensity of the negative control raw data and Ĩ +ve represents the median of the fluorescence intensity of the positive control raw data. Results are summarized in Supplementary Figs S2–S9 . Chemoinformatic analysis The chemotype similarity of every compound compared to each other was determined using shape Tanimoto scores. Shape Tanimoto scores were calculated by Instant JChem (JChem 5.8.0, 2012, ChemAxon, http://www.chemaxon.com ). Chemical substructures of the top eight small molecules ( Fig. 3b ) were generated by NCGC Automatic R-group analysis program (Tripod Development; http://tripod.nih.gov/?p=46 ) [47] . Construction of small molecule microarrays Microarrays were constructed as previously described [20] , [21] , [48] , [49] , [50] , [51] , [52] , [53] , [54] , [55] , [56] . Compounds that were identified as hits from the dye-displacement assay were immobilized onto aldehyde-functionalized microarray via a reductive amination reaction. Serial dilutions of compounds were prepared in 75% DMSO in NANOpure water. A 400-nl aliquot of each serial dilution was then spotted onto the surface (five 1:5 dilutions beginning with 5 mM compound). A negative control for non-specific binding of RNA to the slide surface was generated by delivering 400 nl of 75% DMSO in NANOpure water to the slide surface. The spotted microarray was placed in a humidity chamber for 3 h. The resulting imine was reduced with a solution of 4:1 1× phosphate-buffered saline: ethanol containing 32 mM NaCNBH 3 for 3 min at room temperature. Slides were then washed with 0.1% sodium dodecyl sulfate (SDS; 3×5 min) and water (5×5 min), and allowed to dry to a thin film at room temperature. RNA selection procedures The RNA libraries ( 1 – 3 ) were radioactively labeled by run-off transcription using an RNAMaxx transcription kit (Stratagene). Half the concentration of cold ATP per the manufacturer's protocol and 10 μl of [α- 32 P]ATP (3,000 Ci mol −1 ; Perkin Elmer) were used. Small molecule microarrays were pre-equilibrated with 1× SB2 for 5 min at room temperature. Radioactively labeled internal loop library ( 1 – 3 ; 50 pmol each) and competitor oligonucleotides ( 4 – 8 ; 50 nmol each; Fig. 2 ) were annealed separately in 1× SB1 at 60 °C for 5 min and allowed to slowly cool on the bench top. Folded RNAs were mixed together in a total volume of 400 μl, and BSA was added to a final concentration of 40 μg ml −1 . The mixture was pipetted onto the slide and evenly distributed across the slide surface with a custom-cut sheet of Parafilm. Slides were hybridized at room temperature for 30 min. After the 30-min hybridization period, the slides were washed by submersion in 30 ml of 1× SB2 for 30 min with gentle agitation. This step was repeated three times. Excess buffer was removed from the slide surface, and the slides were left to dry on the bench top. The arrays were exposed to a phosphorimager screen and imaged using a Typhoon 9410 variable mode imager. The image was used as a template to identify spots that bound RNA and to mechanically remove them from the surface. A 400-nl aliquot of NANOpure water was added to the spot to be excised. After 30 s, excess water was pipetted from the surface (most is absorbed), and the gel at that position was excised. RT–PCR amplification The agarose containing bound RNAs was placed into a thin-walled PCR tube with 16 μl of NANOpure water, 2 μl of 10× RQ DNase I buffer and 2 units of RQ DNase I (Promega). The tube was vortexed, centrifuged for 4 min at 8,000 g and then incubated at 37 °C for 2 h. The reaction was quenched by addition of 2 μl of 10× DNase Stop Solution (Promega), and the sample was incubated at 65 °C for 10 min to inactivate the DNase. This solution was used for reverse transcription-PCR (RT–PCR) amplification, which was completed as previously described [57] . Aliquots of the RT–PCR reactions were checked every five cycles starting at cycle 25 on a denaturing 15% polyacrylamide gel stained with ethidium bromide or SYBR Gold (Invitrogen). Multiple rounds of selection The selection procedure was repeated three times with all eight lead small molecules ( PL-1 , HL-1 , HL-2 , HL-3 , HL-4 , DL-1 , DL-2 and DL-3 ) in one spot to enrich the RNA pool. The final round of selection was completed by spotting the small molecules individually as serial dilutions ( Fig. 4 ). Cloning and sequencing The RT–PCR products were cloned into the corresponding site of the pGEM-T vector. Sequencing was completed by Functional Biosciences, Inc. Statistical analysis of selected RNAs Analysis of the selected RNA libraries after multiple rounds of selection was completed by calculating Z obs and P -values. In this analysis, the selected RNAs are compared with the RNAs in the entire starting library. The statistical significance parameter Z obs was then calculated according to equations 2 and 3 (refs 49 , 50 , 51 ): where n 1 is the size of population 1 (the selected RNAs); n 2 is the size of population 2 (the starting library); p 1 is the observed proportion of population 1 (the selected RNAs) that displays the feature of interest; and, p 2 is the observed proportion for population 2 (the starting library) that displays the feature of interest. Z obs is manually converted to the corresponding two-tailed P -value, which represents the confidence level that a feature in the selected RNA sequences is preferred by the ligand and did not occur randomly. The number of RNAs in the starting library and the number of selected RNA sequences are summarized in Supplementary Table S2 . Binding affinity measurements Dissociation constants were determined using an in-solution, fluorescence-based assay [20] , [21] , [48] , [49] , [50] , [51] , [54] , [55] , [58] . A selected RNA or RNA mixture was folded as described above. Then, PL-1 , HL-1 , HL-2 or DL-1 was added to a final concentration of 100, 1,000, 1,000 or 1,000 nM, respectively. Serial dilutions (1:2) were then completed in 1× SB2 containing the corresponding concentration of small molecule. The solutions were incubated for 15 min at room temperature and then transferred to a well of a black 96-well plate. Fluorescence intensity was measured using a Bio-Tek FL×800 plate reader. The change in fluorescence intensity as a function of RNA concentration was fit to the following equation 4 (ref. 59 ): where I is the observed fluorescence intensity; I 0 is the fluorescence intensity in the absence of RNA; Δ is the difference between the fluorescence intensity in the absence of RNA and in the presence of infinite RNA concentration and is in units of M −1 ; [FL] 0 is the concentration of compound; [RNA] 0 is the concentration of the selected RNA; and K t is the dissociation constant. Representative binding curves are shown in Supplementary Figs S22–S28 . How to cite this article: Tran T. and Disney M.D. Identifying the preferred RNA motifs and chemotypes that interact by probing millions of combinations. Nat. Commun. 3:1125 doi: 10.1038/ncomms2119 (2012).